De novobranching cascades for structural and functional diversity in small molecules The limited structural diversity that a compound library represents severely restrains the discovery of bioactive small molecules for medicinal chemistry and chemical biology research, and thus calls for developing new divergent synthetic approaches to structurally diverse and complex scaffolds. Here we present a de novo branching cascades approach wherein simple primary substrates follow different cascade reactions to create various distinct molecular frameworks in a scaffold diversity phase. Later, the scaffold elaboration phase introduces further complexity to the scaffolds by creating a number of chiral centres and incorporating new hetero- or carbocyclic rings. Thus, employing N -phenyl hydroxylamine, dimethyl acetylenedicarboxylate and allene ester as primary substrates, a compound collection of sixty one molecules representing seventeen different scaffolds is built up that delivers a potent tubulin inhibitor, as well as inhibitors of the Hedgehog signalling pathway. This work highlights the immense potential of cascade reactions to deliver compound libraries enriched in structural and functional diversity. Structural diversity has a profound impact on the performance of a compound collection exposed to biological screenings [1] , [2] , [3] . Probe and drug discovery research, therefore, beseech quality-based compound libraries rich in structural diversity [4] , [5] . The latter in turn is primarily determined by the number of diverse scaffolds or chemotypes that represent a compound library [6] , [7] , [8] . Consequently, new synthetic challenges have emerged aiming at divergent access to structurally distinct and complex scaffolds [9] , [10] , [11] . Different approaches have been developed to incorporate structural diversity to a compound collection, for instance, in the build-couple-pair strategies [12] , [13] , folding [14] and branching pathways [15] , [16] , [17] , structural variations either in the building blocks or the reacting partners of common substrates derive the formation of new scaffolds. Synthesis of natural product scaffold-based [18] , [19] , [20] , [21] compound libraries either employs accessible complex natural products or their derivatives for generating new and complex scaffold structures or build up compound libraries around privileged scaffolds [1] , [22] . However, most of the above mentioned synthesis designs require carefully functionalized substrates, as well as their reacting partners and often deliver structural diversity in a compound library at the cost of tedious multistep synthesis protocol. Nature displays it’s amazing ability to assemble a limited pool of simple building blocks into structurally and functionally diverse natural products [23] , [24] . For instance, terpenes that represent a large class of natural products are formally generated from only one biosynthetic unit [25] . Infact, terpenes and sesquiterpenes represent interesting examples of de novo biosynthesis designs where compound collections are generated in two important phases; the first cyclase phase builds up scaffolds from simple acyclic substrates with the help of cyclase enzymes and the next phase elaborates these scaffolds, for instance, with oxidative modifications, to generate a number of diversely functionalized molecules ( Fig. 1a ) [25] , [26] . 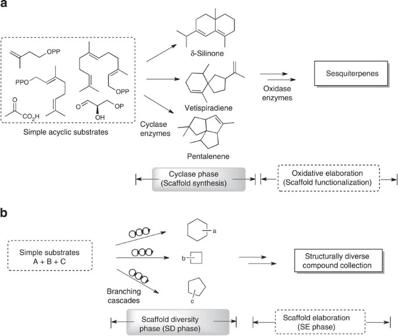Figure 1: Nature’s divergent biogenesis strategy inspires synthetic planning to scaffold diversity. (a) Biogenesis of diverse terpenes from simple substrates; (b) ade novobranching cascades strategy to build a structurally diverse compound collection. Figure 1: Nature’s divergent biogenesis strategy inspires synthetic planning to scaffold diversity. ( a ) Biogenesis of diverse terpenes from simple substrates; ( b ) a de novo branching cascades strategy to build a structurally diverse compound collection. Full size image In contrast to divergent biosynthetic designs, laboratory syntheses targeting diverse scaffolds either choose the substrates already equipped with the ring systems desired in different products or follow multistep and tedious synthetic validations for every target scaffold before producing a library of molecules. Cascade or domino reaction sequences are highly efficient synthetic tools that rapidly build up molecular complexity [27] , [28] . However, their potential in scaffold diversity synthesis remains underexplored. The ‘branching cascades’ strategy is a scaffold diversity synthesis approach wherein common precursors follow different cascade or domino reactions and provide structurally distinct scaffolds for library synthesis [29] . Inspired by the de novo biogenesis of secondary metabolites, we envisioned that the de novo branching cascades could be designed to transform simple acyclic substrates into appreciable scaffold diversity ( Fig. 1b ). In the absence of enzyme weaponry that nature exploits in biogenesis of diverse natural products, the de novo scaffold diversity synthesis with cascade reactions is a formidable synthetic challenge that seeks careful reaction design. Herein we report our efforts towards scaffold diversity synthesis with a de novo branching cascades strategy. Taking cognizance of the biosynthetic library design, we planned to first establish a scaffold diversity phase (SD phase) by transforming simple acyclic substrates into diverse ring systems via branching cascades. While the same set of simple substrates generates different scaffolds, molecular properties like molecular weight and clogP of the resulting distinct scaffolds remain within a threshold limit and can be controlled by small structural variations in the substrates. Therefore, there is a large scope to further modify the generated scaffolds and their appended functionalities in subsequent scaffold elaboration phase (SE phase) and deliver a compound collection rich in structural diversity and molecular complexity ( Fig. 1b ). To establish the principle, a de novo cascade reaction design is chosen in which simple acyclic substrates, N -phenylhydroxylamine, acetylenedicarboxylates and allene esters undergo branching cascades reactions under different reaction conditions to provide seven distinct scaffolds in SD phase. Four of these scaffolds are further elaborated in SE phase to yield a collection of 61 molecules spread over 17 molecular frameworks. Cell-based screenings identify potent and novel bioactive molecules, representing four different structural classes, as inhibitors of tubulin polymerization or hedgehog signalling, and thereby validate the notion that functional diversity is bequeathed to a compound collection by scaffold diversity. Planning of the de novo branching cascades approach Targeting a compound collection of diverse azaheterocycles and employing simple substrates lacking any azaring system, we focused on a cascade reaction sequence that could provide a suitable point of divergence, that is, an intermediate that could be transformed into distinct chemotypes (azaheterocycles) by merely modulating the reaction conditions. N -phenyl nitrones ( 1 ) undergo [3+2] cycloadditions with allenic esters ( 2 ) and the corresponding isoxazolidines ( 3 ) follow a pericyclic rearrangement leading to azepinones ( 5 , Fig. 2 ) [30] , [31] , [32] , [33] , [34] . Azepinone 5 beholds different reactive functionalities like a secondary amine and a β-ketoester that can be exploited in branching cascade approach to build distinct azaheterocyclic frameworks. Moreover, similar azepinones are known to rearrange and yield vinyl indoles ( 6 ) [35] . Cascade reaction sequences, thus, can be designed to explore various reactive functionalities in either the azepinone 5 or vinyl indole 6 to generate new and distinct scaffolds ( Fig. 2 ). 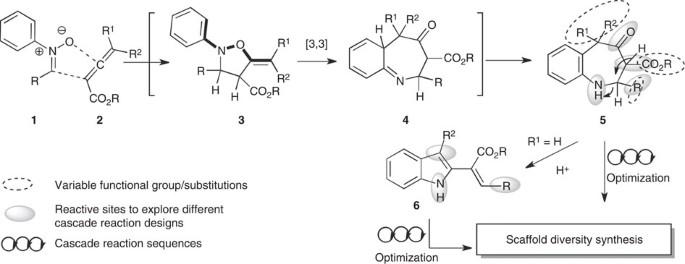Figure 2: A cascade reaction design to explore thede novobranching cascades approach. The key intermediates, azepinone (5) and vinyl indole (6) that could be transformed into structurally distinct molecular frameworks under cascade reaction conditions. Figure 2: A cascade reaction design to explore the de novo branching cascades approach. The key intermediates, azepinone ( 5 ) and vinyl indole ( 6 ) that could be transformed into structurally distinct molecular frameworks under cascade reaction conditions. Full size image Scaffold diversity phase With this planning, reaction conditions were optimized ( Supplementary Table 1 ) for an in situ generation of the nitrone ( 10 ) by addition of phenyl hydroxylamine ( 7 ) to dimethyl acetylenedicarboxylate (DMAD) ( 8 ), and followed by a [3+2] cycloaddition with allene ester ( 2 ), leading to azepinone 11 ( de novo cascade I, Fig. 3a ). DMAD facilitates in situ generation of nitrone [36] , [37] 10 and provides reactive functionalities to build new ring systems in SD phase, as well as to elaborate scaffolds later in SE phase. 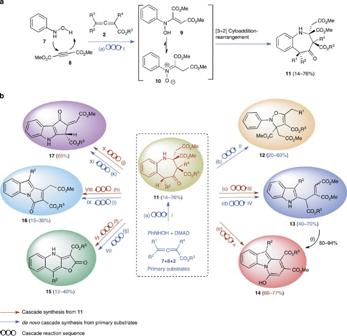Figure 3: Building scaffold diversity phase (SD phase) byde novobranching cascades. (a) Cascade synthesis of azepinone11from primary substrates. (b) SD phase;de novobranching cascades from primary substrates (blue arrows) and branching cascades from azepinone (red arrows) leading to diverse scaffolds, for details seeSupplementary Methods. (a)7+8in MeCN, 10 min, room temperature (RT), then2, 80 °C, 8 h, 14–76%; (b)7+8in MeCN, 10 min, RT, then2, RT, 8 h, 20–60%; (c) TFA (20 mol%) in toluene, 100 °C, 6 h, 60–89%; (d)7+8in MeCN, 10 min, RT, then2, 80 °C, 8 h, then TFA (20 mol%) in toluene, 100 °C, 6 h, 40–70%; (e) TFA (20 mol%) in toluene, 100 °C, 6 h, then NaOH(aq) 1 M, 1,4-dioxane, RT, 6 h and neutralization with HCl (3 M) until pH=6–7, 66–77%; (f) K2CO3, DMF, 100 °C, 6 h, 25–76%; (g)7+8in DMF, 10 min, RT, then2, 80 °C, 8 h, then K2CO3, 100 °C, 6 h, 12–40%; (h) KOAc, EtOH, 60 °C, 6 h, 69% or K2CO3, DMF, 100 °C, 6 h, 15–32%; (i)7+8in DMF, 10 min, RT, then2, 80 °C, 8 h, then K2CO3, 100 °C, 6 h, 15–30%; (j) NaH, DMF, 0 °C, 30 min, 65%; (k)7+8in DMF, 10 min, RT, then2, 80 °C, 8 h, then KOAc, EtOH, 60 °C, 4%; and (l) NaOH(aq) 1 M, 1,4-dioxane, RT, 6 h and neutralization with HCl 3 M until pH=6–7, 80–94%. Figure 3 depicts building of SD phase in a de novo branching cascades approach from primary substrates (indicated by blue arrows), as well as from 11 (indicated by red arrows). Formation of scaffolds 13–17 from azepinone 11 not only confirmed its intermediacy in different cascade reaction sequences, but also provided an efficient access to scaffolds 14 and 17 , which were rather difficult to access directly from primary substrates ( Fig. 3b ). Figure 3: Building scaffold diversity phase (SD phase) by de novo branching cascades. ( a ) Cascade synthesis of azepinone 11 from primary substrates. ( b ) SD phase; de novo branching cascades from primary substrates (blue arrows) and branching cascades from azepinone (red arrows) leading to diverse scaffolds, for details see Supplementary Methods . (a) 7 + 8 in MeCN, 10 min, room temperature (RT), then 2 , 80 °C, 8 h, 14–76%; (b) 7 + 8 in MeCN, 10 min, RT, then 2 , RT, 8 h, 20–60%; (c) TFA (20 mol%) in toluene, 100 °C, 6 h, 60–89%; (d) 7 + 8 in MeCN, 10 min, RT, then 2 , 80 °C, 8 h, then TFA (20 mol%) in toluene, 100 °C, 6 h, 40–70%; (e) TFA (20 mol%) in toluene, 100 °C, 6 h, then NaOH(aq) 1 M, 1,4-dioxane, RT, 6 h and neutralization with HCl (3 M) until pH=6–7, 66–77%; (f) K 2 CO 3 , DMF, 100 °C, 6 h, 25–76%; (g) 7 + 8 in DMF, 10 min, RT, then 2 , 80 °C, 8 h, then K 2 CO 3 , 100 °C, 6 h, 12–40%; (h) KOAc, EtOH, 60 °C, 6 h, 69% or K 2 CO 3 , DMF, 100 °C, 6 h, 15–32%; (i) 7 + 8 in DMF, 10 min, RT, then 2 , 80 °C, 8 h, then K 2 CO 3 , 100 °C, 6 h, 15–30%; (j) NaH, DMF, 0 °C, 30 min, 65%; (k) 7 + 8 in DMF, 10 min, RT, then 2 , 80 °C, 8 h, then KOAc, EtOH, 60 °C, 4%; and ( l ) NaOH(aq) 1 M, 1,4-dioxane, RT, 6 h and neutralization with HCl 3 M until pH=6–7, 80–94%. Full size image Azepinone 11 itself is an interesting scaffold rich in sp 3 character. Using differently substituted allene esters ( 2 ), the first cascade reaction sequence (cascade I) under optimized reaction conditions ( Supplementary Table 1 ) delivered highly substituted azepinones ( 11a–o) . Except for the α-substituted allene esters, which provided 11n–o (R 4 =Me and prenyl) with two consecutive quaternary centres in low yields, azepinones 11a–m were obtained in moderate to high yields (40–76%; Fig. 3b ; Supplementary Fig. 1 ). Interestingly, just changing the reaction condition in cascade I from 80 °C to room temperature provided a different scaffold 12 , that is, a dihydroisoxazole (cascade II; Fig. 3b ; Supplementary Fig. 1 ). To find suitable reaction conditions that could transform the primary substrates into diverse scaffolds via azepinone as intermediate, 11a (R 1 –R 2 , R 4 =H, R 3 =Et) was screened against different Lewis and Brønsted acids. While Lewis acids like BF 3 .OEt 2 or TMSOTf provided only fragmentation products of the azepinone, AlCl 3 yielded an inseparable complex mixture of products ( Supplementary Table 2 ). In a successful case (cascade III), catalytic trifluoroacetic acid (TFA) transformed azepinone 11a into allyl indole ( 13a ; Fig. 3b ) at high temperature (100 °C). After slight modification in this reaction condition, we were able to synthesize allyl indole 13 directly from primary substrates (cascade IV; Fig. 3b ). Allyl indole 13 supports an electron-poor olefin appended to an electron-rich indole, and therefore is a potential building block for higher-order polycyclic indoles. This opportunity was realized by overnight heating of azepinones 11 in toluene with 20 mol% of TFA that would have led to allyl indole ( 13 ), and followed by treatment with sodium hydroxide (NaOH) at room temperature in dioxane that provided us benzo[ b ]indolizine molecules ( 14 ) embodying a naturally occurring scaffold [38] , [39] in high yields (cascade V; Fig. 3b ). In a separate reaction, treatment of allyl indoles 13 with 1 M NaOH also yielded benzo[ b ]indolizines 14 in excellent yields (80–94%). However, attempts to develop a de novo access to 14 directly from primary substrates ( 2 + 7 + 8 ) did not succeed in this case. Azepinone 11 contains more than one nucleophilic site in proximity to different carbonyl functions. Therefore, various modes of cyclization and/or ring-distortion reactions can be realized in the presence of a suitable base, leading to different heterocyclic systems. With this hope, we resorted to a reaction screen of azepinone 11a employing various bases and in different solvents ( Supplementary Table 3 ). The reaction screening revealed various levels of reaction control, that is, effects of different reagents, solvents and temperature in directing substrates to follow a preferred reaction sequence among many possible pathways. For instance, overnight stirring of 11a with potassium carbonate in dimethylformamide (DMF) at room temperature provided a novel scaffold 15 as the only product in low yield (<15%). Increasing the temperature (100 °C) led to the formation of 15 along with another scaffold 16 in appreciable yields. While some other bases attempted in the reaction screening either led to incomplete reactions or heavy decomposition ( Supplementary Table 3 ), this reaction condition was adapted in de novo cascade synthesis from primary substrates delivering substituted scaffolds 15 and 16 in acceptable yields (cascades VII and IX; Fig. 3b ; Supplementary Table 3 ). To our delight, treatment of azepinone 11a ((R 1 –R 2 , R 4 =H, R 3 =Et) with NaH in DMF at 0 °C (decomposition at room temperature) yielded another novel scaffold 17 in high yield (65%, cascade X). Compound 17 embodies an indole-fused cyclopentanone supporting an exocyclic olefin ( Fig. 3b ) that apparently infers C3-indole cyclization to one of the ester function derived from DMAD. Unfortunately, the corresponding de novo synthesis of 17 from primary substrates was very low yielding (4% via cascade XI) and could not be improved. Overall, the de novo branching cascades successfully delivered five scaffolds ( 11–13 and 15–16 ) and two ( 14 and 17 ) were obtained from azepinone 11 . A compound collection of 46 molecules was thus generated in the SD phase ( Supplementary Fig. 1 ). The proposed reaction mechanisms for the de novo cascades I, II and IV leading to the formation of azepinones 11 , isoxazolidines ( 12 ) or allyl indoles ( 13 , Fig. 4a ), respectively, are supported by various reported cycloaddition reactions between N -phenyl nitrones and allenes [30] , [31] , [32] . Notably, de novo cascade II to 12 does not pass through azepinone and the initial [3+2] cycloadducts 18 ( Fig. 4a ) preferred energetically favoured olefinic isomerization to 12 over a sigmatropic rearrangement to azepinone 11 that requires higher temperature. Formation of allyl indoles ( 13 ) apparently occurs via isomerization of vinyl indoles ( 20 ) formed from 11 under optimized reaction conditions ( Fig. 4a ). Benzo[ b ]indolizines ( 14 ) were synthesized under the reaction conditions that first generate an allyl indole 13 , which cyclizes on treatment with a base to yield 14 (cascade V; Fig. 4a ). Although we also expected the formation of scaffold 21 by N -indole cyclization to C2-ester in allyl indoles 13 , however, no trace of 21 was detected ( Fig. 4a ). 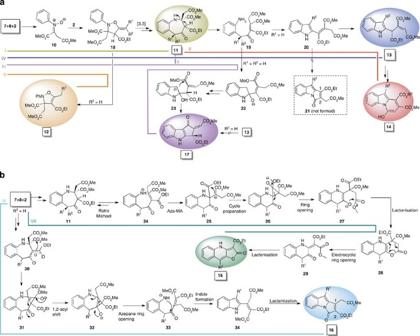Figure 4: Proposed cascade routes to diverse scaffolds in SD phase. (a) Mechanistic proposal for the cascade synthesis of scaffolds11–14,17and (b) for15–16. Compound numbers shown in boxes depict isolated molecules. Differently coloured thick bars display different cascade reaction sequences leading to diverse scaffolds in SD phase. Figure 4: Proposed cascade routes to diverse scaffolds in SD phase. ( a ) Mechanistic proposal for the cascade synthesis of scaffolds 11 – 14 , 17 and ( b ) for 15 – 16 . Compound numbers shown in boxes depict isolated molecules. Differently coloured thick bars display different cascade reaction sequences leading to diverse scaffolds in SD phase. Full size image Structural features of 17 (formed under basic reaction conditions from 11 ) were suggestive of a C3-indole cyclization to one of the ester moieties in allyl indole 13 . However, treatment of 13 with NaH in a separate reaction did not yield indolocyclopentanone 17 ( Fig. 4a ). We assume that treatment of 11 with NaH generates a benzylic anion ( 23 ) via vinylic aminal 22 that adds to one of the esters regioselectively before aromatizing to yield 17 ( Fig. 4a , cascade XI). Formation of scaffolds 15 and 16 (for X-ray analysis see Supplementary Figs 9–10 ) was rather unexpected. For the synthesis of 15 ( cascade VII; Fig. 4b ), we propose that azepinone 11 undergoes a retro-Michael reaction generating an anilide 24 that adds to highly electron-poor Michael acceptor in 24 to give an enolate intermediate 25 . Addition of enolate to ethyl ester moiety generates a cyclopropane that opens concomitantly leading to formation of enolate 27 that cyclizes to form tricyclic lactone 28 . Electrocyclic ring opening in the latter forms the benzylic vinylogous amide 29 that enolizes under basic reaction conditions and cyclizes to provide the scaffold 15 . Scaffold 21 (expected but not formed) and 16 are structurally similar but support the ester and methyl acetate functions (arising from allene ester and DMAD, respectively) on different positions ( Fig. 4a,b ). Mechanistically, we assume that addition of enolate in 30 to the methyl ester on the quaternary centre generates the intermediate 31 that undergoes 1,2-acyl shift to yield anionic malenoate 32 . Ketone formation followed by concomitant cyclopropane and azepane ring opening forms anilide 33 that condenses with keto moiety to form vinyl indole 34 . N -indole cyclization in 34 then generates the final adducts 16 (cascade IX; Fig. 4b ). Scaffold elaboration phase The de novo cascade reactions were designed to adorn scaffolds in SD phase with functional groups that can be exploited to accomplish further complex scaffolds in terms of embodying ring systems, percentage of sp 3 carbons and number of chiral centres, and thus furnishing greater structural diversity to the library. To provide a proof of this principle, we chose four scaffolds generated by de novo cascade design, including structurally flat scaffolds ( 15 – 16 ) for structural elaboration in SE phase ( Fig. 5 ). Following simple one-step transformations, azepinone 11 delivered further complex benzazepane scaffolds 35 – 37 . Treatment of 11 with ammonium fluoride yielded azepinamine 35 . To our delight, two different chemo- and diastereoselective reductions of phenacetone in 11 provided hydroxyl azepane 36 supporting three consecutive chiral centres in high yield and a tricyclic benzazepane lactone 37 that was isolated in low yield as single diastereoisomers ( Fig. 5 ). 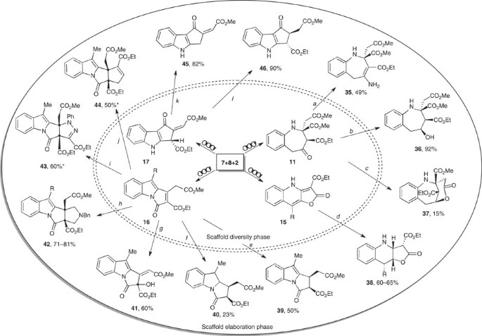Figure 5: SD and SE phases inde novobranching cascades strategy. For details, seeSupplementary Methods. (a) NH4F, MeOH, room temperature (RT), 8 h, 49%; (b) BH3-morpholine, toluene, RT, 6 h, 92% (single diastereomer); (c) DIBAL-H 1.0 M, DCM, from −78 °C to 0 °C, 1 h, 15% (single diastereomer); (d) Na, NH3(liq), THF, −78 °C, 15 min, 60–65% (dr=2.3–4.0:1); (e) 1 bar H2, MeOH, RT, Pd-C, 50% of39(single diastereomer); (f) 8 bar H2, MeOH, RT, Pd-C, 34% of39and 23% of40(dr=4.9:1); (g) Oxone, K2CO3, MeCN-H2O, RT, 1 h, 60% (single diastereomer); (h)N-Methoxymethyl-N-(trimethylsilylmethyl)benzylamine, TFA (1.2 eqv.), toluene, RT, 8 h, 71–81% (single diastereomer for42a); (i) Hydrazonoyl chloride, TEA (2.0 eqv.), toluene, 70 °C, 8 h, 60% (*brsm, single diastereomer); (j) allene ester (2a), tris(4-methoxyphenyl)-phosphine (40 mol%), toluene, RT, 8 h, 50% (*brsm, single diastereomer); (k) TEA(3.5 eqv.), toluene, reflux, 8 h, 82% (E:Z=1:4); and (l) 1 bar H2, Pd-C, MeOH, RT, 12 h, 90% (single diastereomer). Dots in41–44mark the new quaternary centres generated from scaffold16. Figure 5: SD and SE phases in de novo branching cascades strategy. For details, see Supplementary Methods . (a) NH 4 F, MeOH, room temperature (RT), 8 h, 49%; (b) BH 3 -morpholine, toluene, RT, 6 h, 92% (single diastereomer); (c) DIBAL-H 1.0 M, DCM, from −78 °C to 0 °C, 1 h, 15% (single diastereomer); (d) Na, NH 3(liq) , THF, −78 °C, 15 min, 60–65% (dr=2.3–4.0:1); (e) 1 bar H 2 , MeOH, RT, Pd-C, 50% of 39 (single diastereomer); (f) 8 bar H 2 , MeOH, RT, Pd-C, 34% of 39 and 23% of 40 (dr=4.9:1); (g) Oxone, K 2 CO 3 , MeCN-H 2 O, RT, 1 h, 60% (single diastereomer); (h) N -Methoxymethyl- N -(trimethylsilylmethyl)benzylamine, TFA (1.2 eqv. ), toluene, RT, 8 h, 71–81% (single diastereomer for 42a ); (i) Hydrazonoyl chloride, TEA (2.0 eqv. ), toluene, 70 °C, 8 h, 60% (*brsm, single diastereomer); (j) allene ester ( 2a ), tris(4-methoxyphenyl)-phosphine (40 mol%), toluene, RT, 8 h, 50% (*brsm, single diastereomer); (k) TEA(3.5 eqv. ), toluene, reflux, 8 h, 82% ( E : Z =1:4); and (l) 1 bar H 2 , Pd-C, MeOH, RT, 12 h, 90% (single diastereomer). Dots in 41 – 44 mark the new quaternary centres generated from scaffold 16 . Full size image Birch reduction transformed the novel but flat scaffold 15 into sp 3 -rich framework 38 in high yields ( Supplementary Fig. 1 ). Another flat but novel scaffold 16 was transformed into six distinct scaffolds 39 – 44 carrying greater sp 3 character and number of chiral centres ( Fig. 5 ). A stereoselective palladium catalysed hydrogenation of 16 yielded single diastereoisomer of 1,2-dihydro-3 H -pyrrolo[1,2- a ]indol-3-one ( 39 ). Employing higher pressure of the hydrogen in this reaction provided, along with 39 , another sp 3 -rich scaffold, tetrahydro-3 H -pyrrolo[1,2- a ]indol-3-one ( 40 ), although as a mixture of diastereomers (dr~5:1, Fig. 5 ). Oxidation of 16 with oxone-generated scaffold 41 presumably via an intermediary epoxide that opened up under basic condition affording Z - 41 as single diastereomer in high yield ( Fig. 5 , see Supplementary Fig. 53 for the nuclear overhauser effect spectroscopy (NOESY) experiment to confirm relative stereochemistry in 41 ). Scaffold 16 beholds a tetrasubstituted electron-poor olefin that might be explored in different cycloaddition/annulation reactions and could generate two consecutive quaternary centres. However, tetrasubstituted olefins could provide steric resistance to reacting partners. Gratifyingly, scaffold 16 proved to be a nice dipolarophile for various dipolar cycloaddition reactions. A dipolar cycloaddition of 16 with an in situ generated azomethine ylide from N -methoxymethyl- N -(trimethylsilylmethyl)benzylamine [40] led to tetracyclic indole scaffold 42 in high yields (71–81%) and with excellent stereoselectivity. Another in situ generated dipole, the nitrile iminoester [41] , in a low conversion reaction with 16 afforded cycloadduct 43 in a complete regio- and stereoselective manner. Phosphine-catalysed [3+2] cycloaddition of 16 with the zwitterion generated from allene ester ( 2 , R 1 –R 2 , R 4 =H, R 3 =Et) went smoothly and in a regio- and stereoselective manner to provide adduct 44 in moderate yield ( Fig. 5 ) [42] . Notably, this phosphine-catalysed transformation is among the rare cases of dipolar annulations of allene-derived zwitterions with tetrasubstituted olefins [43] , [44] . All cycloadducts formed in above cases, that is, 42 – 44 behold two consecutive quaternary chiral centres. Elaboration of the fourth scaffold 17 involved a base-mediated selective decarboxylation to yield scaffold 45 and a Pd-catalysed hydrogenation to yield scaffold 46 as a single diastereoisomer in excellent yields ( Fig. 5 ). Functional groups like esters or amines present in the scaffolds from SD and SE phases can be utilized to generate a suitable number of compounds adequately representing each scaffold in the compound library. Scaffold diversity and molecular properties analysis Scaffold diversity synthesis outlined in Figures 3 and 5 provided a collection of 61 molecules based on 17 distinct molecular frameworks ( Fig. 6a ; Supplementary Fig. 1 ). Unlike the conventional multistep synthesis of the complex molecules, each distinct scaffold in SD and SE phases was a one-step product that could be easily purified by silica gel column chromatography providing molecules in sufficient amounts for a wide range of biological screenings (see Supplementary Methods ). Some of the cascade reactions in SD phase were performed at 1–2-g scale providing enough amounts of scaffolds for further elaborations. For instance, de novo cascades I, VII and IX provided differently substituted 11 , 15 and 16 in appreciable yields (18–76%) at 1–2-g scale. The fact that no combinatorial synthesis step such as amide synthesis, reductive aminations or coupling reactions etc. were applied to the scaffolds, the potential to build a large and structurally diverse library with this approach is remarkably high. 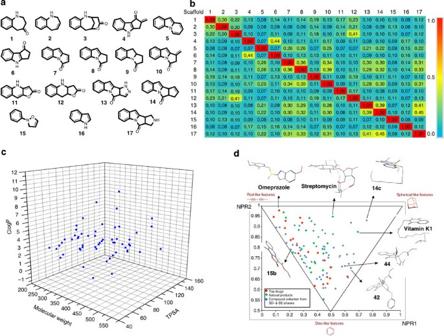Figure 6: Diversity and molecular properties analysis of compounds created in SD and SE phases byde novobranching cascades approach. (a) Structures of 17 diverse scaffolds that make up the core frameworks in the compound collection. (b) Relative tanimoto similarity coefficients for 17 scaffolds (1.0 represents perfect similarity and 0.0 totally distinct scaffolds), for a tanimoto-matrix analysis with different connectivity (seeSupplementary Fig. 2). (c) Molecular properties of the compounds generated in SD and SE phases. (d) Principal moment of inertia (PMI) plot. The molecular shape of the compounds generated in SD and SE phases with branching cascade approach (blue squares) and comparison with 20 natural products (green square) and 20 drugs (red squares). Figure 6: Diversity and molecular properties analysis of compounds created in SD and SE phases by de novo branching cascades approach. ( a ) Structures of 17 diverse scaffolds that make up the core frameworks in the compound collection. ( b ) Relative tanimoto similarity coefficients for 17 scaffolds (1.0 represents perfect similarity and 0.0 totally distinct scaffolds), for a tanimoto-matrix analysis with different connectivity (see Supplementary Fig. 2 ). ( c ) Molecular properties of the compounds generated in SD and SE phases. ( d ) Principal moment of inertia (PMI) plot. The molecular shape of the compounds generated in SD and SE phases with branching cascade approach (blue squares) and comparison with 20 natural products (green square) and 20 drugs (red squares). Full size image Although the molecular architectures of the 17 scaffolds in this compound collection are clearly distinctive, the scaffold diversity was quantified by applying similarity metrics to 17 Bemis–Murcko frameworks ( Fig. 6a ) [45] . To this end, Tanimoto coefficients [46] were generated using extended connectivity fingerprints (ECFP_6, for further details see Supplementary Fig. 2 ) [47] . Figure 6b clearly depicts that most of the 17 scaffolds are largely distinct from one another (from 1.0 to 0, 1.0 for being the same scaffold). Moreover, the compound collection is represented by ring systems found in natural products, drugs and some unprecedented azaheterocycles, and thus covers biologically relevant as well as novel chemical space. Substitutions on substrates directly influence the physical properties of library members. In the de novo branching cascade approach, simple acyclic and low molecular weight substrates provide scaffold diversity, and thereby keep an inherent check over physical properties of the library members. A major portion of the generated library possesses molecular properties within Lipinski’s limits [48] as far as molecular weight, polar surface area and clog P values are concerned. The only molecules that were generated from allene esters supporting lipophilic alkyl chains at γ-position displayed the expected deviations ( Fig. 6c ; Supplementary Table 4 ). In branching cascades approach, some of the reaction sequences were apparently directed by low-energy pathways leading to thermodynamically stable aromatic and flat products. Introduction of greater sp 3 character to the library members enhances the chance of a bioactive molecule to specifically interact with a protein target. Therefore, structural elaboration of the flat scaffolds in SE phase is highly significant. We observed that transition from SD phase to SE phase on average reduced the clog P value by 16% and enhanced the fraction of sp 3 -hybridized carbons (Fsp3) value by >50% ( Supplementary Fig. 3 ) [49] , thereby supporting the elaboration of primary scaffolds into more complex frameworks that deliver bioactive molecules ( Supplementary Fig. 4 ). Principal moment of inertia (PMI) analysis of the lowest-energy conformations of library members, selected natural products and available drugs ( Fig. 6d ; Supplementary Fig. 5 ) was performed to compare their three-dimensional shape diversity [50] . The selected natural products and drugs include a number of well-known substances (for example, Taxol, Penicillin and etc. ), as well as molecules embodying scaffolds similar to those presented in the SD and SE phases. The library members appeared to cover a large area from the central towards the rod-disc side of the triangle quite in a similar manner to biologically active natural products and drug molecules ( Fig. 6d ; for details see Supplementary Figs 6 and 7 and Supplementary Tables 5–7 ). Biological evaluation Scaffold diversity in a compound collection is expected to bestow the molecules’ ability to modulate different biological functions, and thereby sets a platform for medicinal chemistry and probe discovery research projects. To investigate this possibility, the compound collection was screened in two cell-based assays. In the first case, molecules were subjected to a high-content screen that monitors changes in cytoskeleton and DNA in the human cervical carcinoma HeLa cell line [51] . Treatment of cells with compounds at a concentration of 30 μM for 24 h and subsequent staining of DNA, actin filaments and microtubules revealed structurally similar molecules 17 and 45 causing the cells to round up as if they were entering mitosis ( Supplementary Figs 11 and 12 ). The phenotype caused by 17 was similar to that of nocodazole, a known microtubule destabilizer. Mitotic accumulation induced by 17 was further confirmed by a concentration-dependent increase in the percentage of mitotic HeLa cells that were stained for the mitotic marker phospho-histone H3 (see Fig. 7a and Supplementary Fig. 13 ). Treatment with 17 and 45 for 48 h reduced the viability of HeLa cells with similar half-maximal inhibitory concentrations (IC 50 ) of 3.87±0.01 μM and 3.86±0.77 μM, respectively ( Supplementary Fig. 14 ). Live-cell imaging of HeLa cells treated with 2.5 μM 17 demonstrated that cells were arrested in mitosis for several hours before undergoing apoptosis as detected by membrane blebbing and cell shrinkage ( Supplementary Movies 1–3 ). 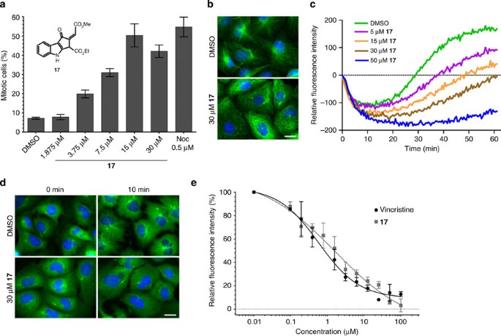Figure 7: Influence of17on HeLa cells and microtubules. (a)17induces mitotic arrest. HeLa cells were treated for 24 h with different concentrations of17or DMSO and nocodazole (Noc) as controls. Cells were then fixed and stained for DNA, the mitotic marker phospho-histone H3 and tubulin. High-content analysis was performed to determine the percentage of mitotic cells using the MetaMorph software. Data are shown as mean values (n=3)±s.d. (b)17impairs the microtubule cytoskeleton in HeLa cells. Cells were treated with 10 μM17or DMSO for 2 h. After fixation, cells were stained for tubulin and DNA using an anti-tubulin antibody coupled to FITC (green) and DAPI (blue), respectively. Scale bar, 20 μm. (c)17inhibits tubulin polymerizationin vitro. Tubulin polymerization was monitored by means of increase of fluorescence intensity of DAPI on binding to microtubules at ex/em 340/460 nm. Data are representative of three independent experiments. (d)17inhibits the regrowth of microtubules in HeLa cells. Cells were treated with 10 μM17and DMSO for 2 h before incubation on ice for 1 h. Cells were rewarmed at 37 °C for given time intervals and then fixed and stained as described inb. Scale bar, 20 μm. Pictures shown are representative of three biological replicates. (e)17displaces BODIPY-FL-vinblastine from tubulin. Porcine brain tubulin was incubated with BODIPY-FL-vinblastine and different concentrations of17or vincristine as a control for 40 min at 25 °C. Fluorescence intensity was then monitored at ex/em 470/514 nm. Decrease in fluorescence indicates competition with BODIPY-FL-vinblastine for binding to the vinca-binding site. Data are shown as mean values (n=3)±s.d. and were normalized to DMSO. Figure 7: Influence of 17 on HeLa cells and microtubules. ( a ) 17 induces mitotic arrest. HeLa cells were treated for 24 h with different concentrations of 17 or DMSO and nocodazole (Noc) as controls. Cells were then fixed and stained for DNA, the mitotic marker phospho-histone H3 and tubulin. High-content analysis was performed to determine the percentage of mitotic cells using the MetaMorph software. Data are shown as mean values ( n =3)±s.d. ( b ) 17 impairs the microtubule cytoskeleton in HeLa cells. Cells were treated with 10 μM 17 or DMSO for 2 h. After fixation, cells were stained for tubulin and DNA using an anti-tubulin antibody coupled to FITC (green) and DAPI (blue), respectively. Scale bar, 20 μm. ( c ) 17 inhibits tubulin polymerization in vitro . Tubulin polymerization was monitored by means of increase of fluorescence intensity of DAPI on binding to microtubules at ex/em 340/460 nm. Data are representative of three independent experiments. ( d ) 17 inhibits the regrowth of microtubules in HeLa cells. Cells were treated with 10 μM 17 and DMSO for 2 h before incubation on ice for 1 h. Cells were rewarmed at 37 °C for given time intervals and then fixed and stained as described in b . Scale bar, 20 μm. Pictures shown are representative of three biological replicates. ( e ) 17 displaces BODIPY-FL-vinblastine from tubulin. Porcine brain tubulin was incubated with BODIPY-FL-vinblastine and different concentrations of 17 or vincristine as a control for 40 min at 25 °C. Fluorescence intensity was then monitored at ex/em 470/514 nm. Decrease in fluorescence indicates competition with BODIPY-FL-vinblastine for binding to the vinca-binding site. Data are shown as mean values ( n =3)±s.d. and were normalized to DMSO. Full size image A closer look at the influence of 17 (10 μM), which is a more functionalized analogue of 45 , on the cytoskeleton in interphase cells revealed a disorganization of the microtubule network already after 2 h of treatment ( Fig. 7b ). In contrast to control cells wherein microtubules emerged from the microtubule organizing centre (MTOC) near the nucleus (visible as the most intense tubulin staining) and extend towards the cell periphery, microtubules in 17 (10 μM)-treated HeLa cells did not converge in the MTOC and their radial organization was distorted. Microtubules are highly dynamic structures that are important for the maintenance of cell shape, inner cellular transport and cell division [52] , and remain an attractive target for anticancer treatment [52] , [53] . The influence of 17 on microtubule dynamics was investigated in vitro using porcine brain tubulin. A concentration-dependent inhibition of tubulin polymerization was monitored by means of the increase of 4′,6-diamidino-2-phenylindole (DAPI) fluorescence on binding to microtubules ( Fig. 7c ) [54] . 17 also inhibited the polymerization of microtubules in HeLa cells after cold treatment ( Fig. 7d ; Supplementary Fig. 15 ). Microtubules reversibly disintegrate at low temperatures and their repolymerization can be monitored after rewarming cells to 37 °C. While in dimethylsulphoxide (DMSO)-treated cells, microtubules started to repolymerize 2 min after rewarming, and nearly complete reconstitution of the mictrotubule cytoskeleton was observed after 10 min, in HeLa cells treated with 10 μM solution of 17 , no regrowth of microtubules was detected even 10 min after rewarming. Thus, 17 is a novel microtubule destabilizing small molecule [55] . Among the three well-characterized binding sites in tubulin, tubulin destabilizers bind to either colchicine or vinca alkaloid-binding sites. Binding of 17 to these binding sites was assessed by means of competition experiments. On binding to tubulin, the intrinsic fluorescence of colchicine increases and displacement of colchicine by small molecules leads to the decrease in fluorescence as detected for nocodozole ( Supplementary Fig. 16a ) [56] . Unfortunately, due to autofluorescence of 17 , it was not possible to determine a putative influence of the compound on the binding of colchicine to tubulin ( Supplementary Fig. 16b ). However, 17 but not colchicine could displace BODIPY-FL-vinblastine from tubulin in a concentration-dependent manner with a half-maximal effective concentration (EC 50 ) of 0.67±1.51 μM ( Fig. 7e ; Supplementary Fig. 17 ), and thus most likely binds to the vinca site in tubulin. Molecules from SD and SE phases were also subjected to a screen that monitors modulation of Hedgehog signalling. The Hedgehog pathway plays a fundamental role during animal embryonic and post-embryonic development by regulating proliferation, migration and differentiation [53] , [57] . In adults, the pathway is silenced and can be reactivated for tissue repair and regeneration [58] . Moreover, the Hedgehog pathway can be involved in tumorigenesis since aberrant Hedgehog signalling is detected in various cancers [53] , [58] . Therefore, small-molecule modulators of the Hedgehog pathway are highly desired for drug discovery and chemical biology investigations. To find inhibitors of Hedgehog signalling, we employed the pluripotent mesenchymal C3H10T1/2 cells that undergo osteogenic differentiation on activation with Hedgehog ligands or purmorphamine, which in turn is characterized by the expression of alkaline phosphatase (AP) and can be used to monitor Hedgehog signalling [59] , [60] . Screening of the compound collection identified 11b (dr~5:2:1), 15g and 16c as inhibitors of Hedgehog signalling, which dose-dependently decreased AP activity in C3H10T1/2 cells (without influencing cell viability) with IC 50 of 0.79, 0.84 and 0.16 μM, respectively ( Fig. 8a,b ). The high-performance liquid chromatography purified major diastereomer of azepinone 11b (for purification and structural assignment, see Supplementary Methods ) was found to be more potent than the two different isomeric mixtures of 11b employed in the assay ( Supplementary Fig. 18 ). Binding of lipophilic Hedgehog proteins to the transmembrane protein patched 1 (Ptch-1) triggers a signalling cascade by relieving Ptch-1-induced repression of the transmembrane protein Smoothened (Smo). This results in the activation of glioma-associated oncogene homologues (Gli)-dependent transcription of Hedgehog pathway-specific target genes [61] . 11b , 15g and 16c suppressed the expression of the Hedgehog target gene Ptch-1 (ref. 62 ) in NIH/3T3 cells on stimulation with purmorphamine ( Fig. 8c ). Furthermore, all three molecules inhibited the expression of a Gli-responsive luciferase reporter gene in Shh-LIGHT2 cells [63] ( Fig. 8d ). Several Hedgehog inhibitors operate by binding to and inhibiting Smo [64] . However, 11b , 15g and 16c failed to displace BODIPY-cyclopamine from Smo, and thus most likely do not bind to this receptor ( Fig. 8e ; Supplementary Fig. 19 ). As a result, three new structural classes of Hedgehog inhibitors were discovered providing vital starting points in medicinal chemistry research that targets Hedgehog inhibition-based therapeutics. To obtain an acceptable structure activity relationship (SAR), screening of a larger set of molecules is required. Therefore, a conclusive SAR for the Hedgehog inhibition by molecules based on scaffolds 15 and 16 could not be realized (see Supplementary Fig. 4 for results from the primary screen). However, the results of the primary high-throughput screening for Hedgehog inhibition with benazepinones ( 11 ) indicate that the benzylic substitution significantly modulates the bioactivity and prefers methyl and ethyl groups over the bulkier ones ( Supplementary Fig. 4 ). Although 11e (with an ethyl-β-ketoester and an ethyl group on benzylic carbon) appeared to be active in the primary screening, it displayed an IC 50 >10 μM for the inhibition of purmorphamine-induced osteogenesis (data not shown). 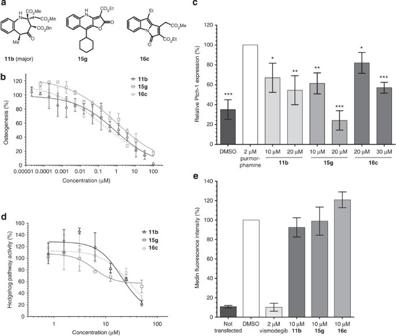Figure 8: Influence of selected compounds on Hedgehog signalling. (a) Chemical structures of11b(structure for the major diastereomer is shown),15gand16c. (b) Influence of11b,15gand16con purmorphamine-induced osteogenesis in C3H10T1/2 cells as determined by the activity of alkaline phosphatase. C3H/10T1/2 cells were treated for 96 h with 1.5 μM purmorphamine and different concentrations of the compounds or DMSO as control. Activity of alkaline phosphatase was determined using a luminescent readout. Nonlinear regression was performed using a four parameter fit. Data are mean values (n=3)±s.d. and were normalized to purmorphamine-treated cells. (c) Influence of11b,15gand16con the relative expression of Ptch-1. NIH/3T3 cells were incubated with 2 μM purmorphamine and different concentrations of the compounds or DMSO as control for 48 h. Following cDNA preparation, the relative expression levels of Ptch-1 and Gapdh were determined by means of quantitative PCR. Data are mean values (n=3)±s.d. and were normalized to purmorphamine-treated cells (*P<0.05, **P<0.01 and ***P<0.001). (d) Influence of11b,15gand16con Gli-mediated reporter gene expression. Shh-LIGHT2 cells were treated with 4 μM purmorphamine and different concentrations of the compounds or DMSO as control for 48 h. Luciferase activity was determined as a measure of Hedgehog pathway activity. Data are mean values (n=3)±s.d. and normalized to cells treated with purmorphamine. (e) Influence of the compounds on the binding of BODIPY-cyclopamine to Smo. HEK293T cells were transfected with a Smo-expression construct. Two days later, cells were treated with the compounds or DMSO as control in the presence of 5 nM BODIPY-cyclopamine for 5 h. Cells were then subjected to flow cytometric analysis to detect Smo-bound BODIPY-cyclopamine. The graph shows the median BODIPY-cyclopamine fluorescence intensity on treatment with the compounds. Data are mean values (n=3)±s.d. Figure 8: Influence of selected compounds on Hedgehog signalling. ( a ) Chemical structures of 11b (structure for the major diastereomer is shown), 15g and 16c . ( b ) Influence of 11b , 15g and 16c on purmorphamine-induced osteogenesis in C3H10T1/2 cells as determined by the activity of alkaline phosphatase. C3H/10T1/2 cells were treated for 96 h with 1.5 μM purmorphamine and different concentrations of the compounds or DMSO as control. Activity of alkaline phosphatase was determined using a luminescent readout. Nonlinear regression was performed using a four parameter fit. Data are mean values ( n =3)±s.d. and were normalized to purmorphamine-treated cells. ( c ) Influence of 11b , 15g and 16c on the relative expression of Ptch-1. NIH/3T3 cells were incubated with 2 μM purmorphamine and different concentrations of the compounds or DMSO as control for 48 h. Following cDNA preparation, the relative expression levels of Ptch-1 and Gapdh were determined by means of quantitative PCR. Data are mean values ( n =3)±s.d. and were normalized to purmorphamine-treated cells (* P <0.05, ** P <0.01 and *** P <0.001). ( d ) Influence of 11b , 15g and 16c on Gli-mediated reporter gene expression. Shh-LIGHT2 cells were treated with 4 μM purmorphamine and different concentrations of the compounds or DMSO as control for 48 h. Luciferase activity was determined as a measure of Hedgehog pathway activity. Data are mean values ( n =3)±s.d. and normalized to cells treated with purmorphamine. ( e ) Influence of the compounds on the binding of BODIPY-cyclopamine to Smo. HEK293T cells were transfected with a Smo-expression construct. Two days later, cells were treated with the compounds or DMSO as control in the presence of 5 nM BODIPY-cyclopamine for 5 h. Cells were then subjected to flow cytometric analysis to detect Smo-bound BODIPY-cyclopamine. The graph shows the median BODIPY-cyclopamine fluorescence intensity on treatment with the compounds. Data are mean values ( n =3)±s.d. Full size image Recent analyses of large data sets of synthetic compounds have indicated that a major part of them is presented by a small percentage of scaffolds and the same is true for drug molecules [65] . The redundancy in the scaffolds representing compound libraries that are used in the discovery research severely restrains the biological scope of the small molecules. Synthetic designs leading to significant scaffold diversity are expected to yield highly useful novel small-molecule candidates for drug and probe discovery research. The de novo branching cascades strategy imbibes inspiration from biogenesis of natural products, employs simple substrates in the reaction designs to generate suitably functionalized scaffolds via cascade reactions and leads to a compound collection rich in scaffold diversity. With just three simple substrates, that is, phenylhydroxylamine, DMAD and allene ester, a collection of 61 molecules represented by 17 scaffolds was generated without employing any combinatorial synthesis step. The structurally diverse compound collection in turn delivered functionally diverse small molecules as potent inhibitors of the tubulin cytoskeleton or the Hedgehog signalling pathway, thus paving the way for their further biological applications. We believe that endeavours to develop divergent access to novel chemical space get more exciting and challenging when driven alongside by chemists’ desire to explore novel chemical reactivity. In fact, many reactive intermediates reported in various cascade or domino reactions including multi-component reactions might be explored in scaffold diversity synthesis and in unravelling new chemical transformations of broader synthetic applications. This work highlights on the one hand, the immense potential of cascade reactions in building structural diversity and molecular complexity from simple substrates and on the other hand validates the notion that functional diversity of a compound collection is a direct consequence of its scaffold diversity. Chemical synthesis Compounds were synthesized according to the procedures specified in Supplementary Methods . X-ray crystallographic data and images are reported in Supplementary Figs 8–10 and Supplementary Tables 8–20 . For 1 H, 13 C and two-dimensional nuclear magnetic resonance spectra of compounds see Supplementary Figs 20–59 ). Scaffold diversity assesment Two different heat maps were generated to assess the scaffold similarity. The calculation was performed using the software PipelinePilot 9.0.2 from the company Accelrys. Calculation based on the ECFP_4 and ECFP_6 (extended connectivity feature-based fingerprint on four and six bonds, respectively; Supplementary Fig. 2 ). Molecular properties were calculated using ChemBioDraw 12.0 software ( Supplementary Table 4 ). Representative values of Fsp3 and clogP for SD phase and SE phase molecules are shown in Supplementary Fig. 3 . PMI calculations We compared the molecular shape diversity of our library with established reference sets of 20 top-selling brand name drugs and 20 diverse natural products ( Supplementary Figs 6 and 7 ). PMI were calculated using Molecular Operating Environment, MOE software package, after minimization of energy of each molecule using a MMFF94x force field with the generalized Born solvation model; eps=r, cutoff [8,10] and gradient=0.1 RMS Kcal mol −1 A −2 . The PMI and related calculations are performed in units of daltons (AMU) and angstroms. The stochastic conformational search algorithm in the MOE software package was used to generate three-dimensional conformers for each compound. Sampling and minimization parameters were implemented as follows: stochastic search limit: 7; refinement conformation limit: 300; stochastic search failure limit: 100; stochastic search iteration limit: 1,000; energy minimization iteration limit: 200; and energy minimization gradient test: 0.01; only the conformer with the lowest energy was retained for PMI calculations in each conformational sampling run ( Supplementary Fig. 5 ; Supplementary Tables 5–7 ). Normalized PMI ratios (I1/I3 and I2/I3) of these conformers were obtained from MOE and then plotted on a triangular graph, with the coordinates (0,1), (0.5,0.5) and (1,1) representing a perfect rod, disc and sphere, respectively, based on the report in ref. 50 . Phenotypic screen HeLa cells were obtained from DSMZ GmbH, Germany and were seeded in black clear bottom 96-well microtiter plates. After incubation overnight, cells were treated with the compounds for 24 h at 30 μM. Cells were fixed with 3.7% formaldehyde in Tris-buffered saline (TBS) and permeabilized with 0.1% Triton X-100 in TBS for 15 min each before blocking using 2% bovine serum albumin (BSA) in TBS/0.1% Tween-20 (TBS-T). Cells were then stained for actin, tubulin and DNA with phalloidin coupled to tetramethylrhodamine, anti-α-tubulin antibody coupled to fluorescein isothiocyanate (FITC) and DAPI, as well as anti-phospho-histone H3 (phospho S10) coupled to AlexaFluor594 (in case of quantification of mitotic cells). Image acquisition was performed on an automated microscope Axiovert M200 (Carl Zeiss, Germany) at 20 × magnification using MetaMorph 7.7.8.0 software (Molecular Devices, USA). Immunocytochemistry After seeding and treatment with compounds, cells were fixed with 3.7% formaldehyde and permeabilized with 0.1% Triton X-100 in TBS. Samples were then blocked with 2% BSA in TBS-T before staining for tubulin and DNA with an anti-α-tubulin antibody coupled to FITC and DAPI, respectively. Axiovert Observer Z1 or Axiovert M200 microscopes (Carl Zeiss) were used for image acquisition. Fluorescence-based tubulin polymerization assay 10 μM Porcine α/β-tubulin (>99% pure, cytoskeleton, USA, in 80 mM Na-PIPES pH 6.9, 1 mM MgCl 2 , 1 mM EGTA and 0.88 mM Na-glutamate) was dissolved in general tubulin buffer containing 16.67% tubulin glycerol buffer, 1 mM GTP and 0.01 mg/ml DAPI on ice. The compound or DMSO were added and fluorescence was measured at 37 °C using the Infinite® M200 plate reader (Tecan, Austria) with excitation/emission wavelengths of 340/460 nm. Microtubule regrowth assay HeLa cells were seeded on cover slips and incubated overnight followed by treatment with 10 μM 17 or DMSO as a control for 2 h. Depolymerization of microtubules was achieved by cold treatment at 4 °C for 1 h. Afterwards, the microtubule cytoskeleton was allowed to repolymerize by placing cells to 37 °C. Cells were fixed in 3.7% formaldehyde in TBS at given intervals before or after rewarming. Microtubules were visualized with an anti-α-tubulin antibody coupled to FITC. DAPI was used to stain DNA. Axiovert Observer microscope Z1 (Carl Zeiss) was used for image acquisition. Colchicine competition assay A 1:2 dilution series of the compound or nocodazole as a control was prepared on ice using a master mix containing 5 mM tubulin (dissolved in general tubulin buffer), 1 mM GTP, 50 μM colchicine, 16.9% v/v tubulin glycerol buffer and 76.6% v/v TR-FRET buffer. After incubation for 40 min at 25 °C, fluorescence intensity was measured in black 96-well plates at ex/em 365/435 nm using the Infinite M200 plate reader (Tecan). Blank values were subtracted from all sample values. Values were normalized to the DMSO control. Vinblastine competition assay A 1:2 dilution series of the compound or vincristine as a control was prepared on ice using a master mix containing 5 mM tubulin (dissolved in general tubulin buffer), 1 mM GTP, 5 μM BODIPY-FL-vinblastine (Invitrogen, Germany), 16.9% v/v tubulin glycerol buffer and 76.6% v/v TR-FRET buffer. After incubation for 40 min at 25 °C, fluorescence intensity was measured in black 96-well plates at ex/em 470/514 nm using the Infinite M200 plate reader (Tecan). Blank values were subtracted from all sample values. Values were normalized to the DMSO control. Osteogenesis C3H10T1/2 cells were obtained from ATCC, USA. Eight hundred C3H/10T1/2 cells were seeded per well in white 384-well plates. On the next day, cells were treated with 1.5 μM purmorphamine and different concentrations of the compounds or DMSO as a control. After 96 h, the luminogenic AP substrate CDP-Star (Roche) was added to the wells to detect AP activity. One hour after addition of CDP-Star, luminescence was measured on an Infinite M200 plate reader (Tecan). Nonlinear regression was performed using a four parameter fit (GraphPad Prism 6, GraphPad Software, La Jolla, California, USA). Quantitative PCR NIH/3T3 cells were obtained from DSMZ GmbH and were seeded in 24-well plates (2 × 10 4 cells per well). After incubation overnight, cells were treated with 2 μM purmorphamine and the compounds or DMSO as a control for 48 h. Complementary DNA (cDNA) was prepared using the FastLane Cell cDNA Kit (Qiagen) following the manufacturer’s instructions. The relative messenger RNA amount of the Hedgehog target gene Ptch-1 and the housekeeping gene Gapdh (glyceraldehyde-3-phosphate dehydrogenase) was assessed using the QuantiFast SYBR Green PCR Kit (Qiagen) and the following primers: 5′-CAGTGCCAGCCTCGTC-3′ and 5′-CAATCTCCACTTTG-CCACTG-3′ for Gapdh; and 5′-CTCTGGAGCAGATTTCCAAGG-3′ and 5′-TGCCGCAGTTCTTTTGAATG-3′ for Ptch-1 (ref. 62 ) The SYBR Green signal was detected with an iQ5 Real-Time PCR Detection System (Bio-Rad, Germany). Expression levels of Ptch-1 were normalized to Gapdh and were related to the expression level of purmorphamine-treated cells. Significance was determined using the unpaired t -test using the GraphPad Prism 6 software (San Diego, USA). Differences were considered statistically significant at P <0.05, confidence interval: 95%. Gli-mediated reporter gene assay For detection of the Gli-mediated reporter gene expression, the reporter cell line Shh-LIGHT2 was employed. Shh-LIGHT2 cells are NIH/3T3 cells, stably transfected with a Gli-responsive firefly luciferase reporter plasmid and a pRL-TK vector for constitutive expression of Renilla luciferase [61] , [63] . Shh-LIGHT2 cells (3.0 × 10 4 ) were seeded per well in 96-well plates. After incubation overnight, cells were treated with 4 μM purmorphamine and the compounds or DMSO as a control for 48 h. Luciferase expression and activity were detected by means of the Dual-Luciferase Reporter Assay System (Promega) using the Infinite M200 plate reader (Tecan). Nonlinear regression was performed using a four parameter fit (GraphPad Prism 6, GraphPad Software). Smoothened-binding assay Flow cytometric analysis of BODIPY-cyclopamine-labelled cells was performed as described in ref. 66 . Briefly, 2.5 × 10 5 HEK293T cells were seeded per well in 6-well plates. After incubation overnight, the cells were transfected with a Smo-expression construct (pGEN-mSmo, a gift from Philip Beachy, Addgene no. 37673) [63] using Fugene HD (Promega). Two days after transfection, cells were treated with the compounds or DMSO in DMEM containing 0.5% FBS and 5 nM BODIPY-cyclopamine (Carbosynth Limited) for 5 h at 37 °C. Cells were then detached and diluted in DMEM containing 0.5% FBS before centrifugation at 129 RCF for 5 min at room temperature. Cells were washed twice in ice-cold PBS and were finally collected by centrifugation at 129 RCF for 5 min at 4 °C. Cells were resuspended in ice-cold PBS and subjected to flow cytometric analysis employing the BD LSR II Flow Cytometer (laser line: 488 nm, emission filter: 530/30) to detect BODIPY. Data were analysed with the FlowJo software, version 7.6.5 (Tree Star Inc., USA) and the Flowing software, version 2.5.1 (by Perttu Terho, University of Turku, Finland/ Turku Bioimaging). Accession codes: The X-ray crystallographic coordinates for structures reported in this article have been deposited at the Cambridge Crytallographic Data Center, under deposition numbers CCDC 943382, 943383 and 943385. These data can be obtained free of charge from Cambridge Crytallographic Data Centre via www.ccdc.cam.ac.uk/data_request/cif . How to cite this article: Garcia-Castro, M. et al. De novo branching cascades for structural and functional diversity in small molecules. Nat. Commun. 6:6516 doi: 10.1038/ncomms7516 (2015).